A functional network perspective on response inhibition and attentional control Inferior frontal cortex (IFC) modules that inhibit dominant behaviours are a popular feature in theories of cognitive dysfunction. However, the paradigms on which these theories are based fail to distinguish between inhibitory and non-inhibitory cognitive demands. Here we use four novel fMRI variants of the classic stop-signal task to test whether the IFC houses unique inhibitory modules. Our results demonstrate that IFC sub-regions are not functionally unique in their sensitivities to inhibitory cognitive demands, but instead form components of spatially distributed networks. These networks are most strongly activated when infrequent stimuli are being processed, regardless of behavioural inhibitory demands, and when novel tasks are being acquired, as opposed to when routine responses must be suppressed. We propose that there are no inhibitory modules within the frontal lobes and that behavioural inhibition is an emergent property of spatially distributed functional networks, each of which supports a broader class of cognitive demands. A major focus in the cognitive neurosciences has been the search for a better understanding of the neural mechanisms underlying behavioural inhibition. This search has been motivated by the fact that impulsivity is a common characteristic of many psychiatric and neurological populations [1] , [2] , [3] , [4] , [5] . A wealth of converging evidence has been reported in support of the view that the frontal lobes make a critical contribution to the performance of behavioural inhibition paradigms; however, the precise nature of those contributions remains divisive [6] , [7] , [8] , [9] , [10] , [11] . Within the impulsivity literature, studies often assume that the frontal lobes house unique neural modules, a sub-set of which are dedicated to the task of inhibiting dominant behaviours. This assumption is based on the observation of heightened frontal lobe activations during the performance of classical inhibitory paradigms such as the stop-signal task (SST) and go/nogo task [12] , [13] . Such observations are reinforced by studies that report differences in the strengths of frontal-lobe activations in clinical populations [1] , [2] , [3] , [4] , [5] or in response to pharmacological interventions [14] , [15] , [16] . Together, these findings have driven a sharp increase in the number of studies that seek to probe ‘inhibitory systems’ using the SST [17] , [18] , [19] , [20] . The right inferior frontal gyrus (RIFG) is the most common candidate for an inhibitory module and is proposed to support reactive inhibition, the transient cancellation of actions when environmental ‘stop signals’ are detected [19] , [21] . More recently, it has been proposed that the right inferior frontal sulcus (RIFS) contains a second inhibitory module that supports proactive inhibition, the sustained downregulation of actions when the requirement to stop is expected [17] , [22] . A major limitation for the inhibitory perspective on frontal-lobe function is that the SST and go/nogo task do not control for potentially confounding non-inhibitory cognitive demands [6] , [7] , [8] , [9] , [10] , [11] , [23] , [24] , [25] . Thus, the common assumption that regional activations during classical inhibitory paradigms ( Fig. 1a ) equate to proof of an involvement in neural inhibitory processes has not been established. Indeed, in the broader literature it has been reported that the RIFG is recruited during a range of attentionally demanding conditions that have no obvious requirement for behavioural inhibition. Notably, these conditions include target detection ( Fig. 1b ) [6] , [26] , [27] , [28] in which the presentation of a target stimulus triggers the initiation as opposed to the cancellation of a motor response. Similarly, the RIFS is recruited during a wide range of cognitive tasks that require the processing of information according to rules, for example, reasoning, planning and mental rotation [7] , [29] , [30] , [31] . Thus, inhibitory theories are overspecified because they do not explain the broader contributions that the putative inhibitory modules make to cognition. 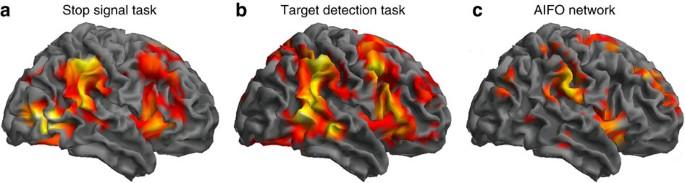Figure 1: Similar right IFG activation across multiple task contexts. (a) Strong activation is evident in the RIFG during performance of the SST (N=81)6. (b) However, a highly similar pattern of activation is evident during target detection, in which there is no dominant response to override (N=14)26. (c) More generally, a spatially very similar, bilateral anterior insula, frontal operculum–anterior cingulate cortical (AIFO–ACC) functional network is strongly recruited during working memory and attentional tasks (N=16)29. All t contrasts rendered withP<0.05, voxel-wise FDR correction for the whole-brain mass. Figure 1: Similar right IFG activation across multiple task contexts. ( a ) Strong activation is evident in the RIFG during performance of the SST ( N =81) [6] . ( b ) However, a highly similar pattern of activation is evident during target detection, in which there is no dominant response to override ( N =14) [26] . ( c ) More generally, a spatially very similar, bilateral anterior insula, frontal operculum–anterior cingulate cortical (AIFO–ACC) functional network is strongly recruited during working memory and attentional tasks ( N =16) [29] . All t contrasts rendered with P <0.05, voxel-wise FDR correction for the whole-brain mass. Full size image Functional connectivity analyses also accord particularly poorly with the modular account of frontal-lobe function, because inferior frontal cortex (IFC) areas typically co-activate with broader cortical networks ( Fig. 1c ) [29] , [32] , [33] , the other components of which respond to similar cognitive demands. These other components include the pre-supplementary motor area (preSMA), which has also been proposed to play a critical role in motor response inhibition [24] , [34] . Consequently, we have proposed that the RIFG and RIFS house sub-components of distributed functional networks as opposed to functionally unique modules [29] . The former network is proposed to support a general class of attentional and working memory maintenance processes, whereas the latter network is proposed to support a general class of reasoning, planning and rule-processing demands. Here we directly test whether sub-components of the human IFC can reasonably be described as inhibitory modules. We apply four novel functional magnetic resonance imaging (fMRI) variants of the classical SST that hold stimulus-processing demands constant while varying proactive-inhibitory, reactive-inhibitory, attentional and rule-processing demands ( Fig. 2 ). Using carefully controlled contrasts, independent components analyses and psychophysiological interactions (PPIs), we test multiple opposing predictions from the reactive inhibition/proactive inhibition (RIPI) account of IFC function [17] and the alternative attentional and rule-processing (ARP) account [6] , [29] . Our results demonstrate that although the IFC is a heterogeneous structure that houses multiple functionally distinct sub-regions, none of these sub-regions is functionally unique within the brain. Moreover, none of these sub-regions responds to inhibitory demands either specifically or even particularly strongly when compared with non-inhibitory task manipulations. 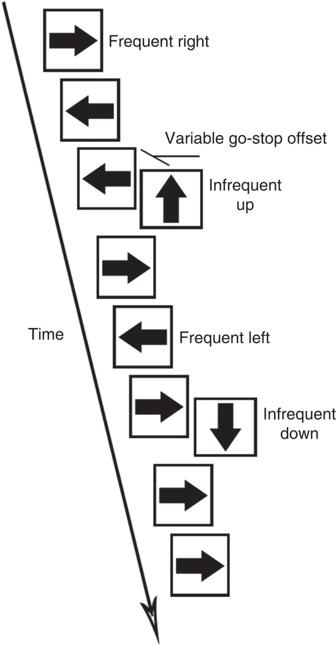Figure 2: Task design. Frequent left and right arrows were displayed with a variable interstimulus interval (1,600, 1,700, 1,800, 1,900 or 2,000 ms). In 91 trials, an infrequent up or down arrow interrupted the frequent stimuli at an unpredictable offset (mean=323 ms, s.d.=122 ms). Each task consisted of 4 × 3 min blocks interleaved with 5 × 40 s of rest. This mixed block-event-related design allowed sustained task-rest activations and transient activations during infrequent−frequent stimuli to be estimated separately. In the MONITOR task, individuals responded to frequent stimuli with a corresponding left or right button press. Participants were instructed to simply monitor the infrequent stimuli. In the INHIBITION task, participants were instructed to respond as fast as they could to the left and right arrows but to try and cancel their response if an up or down arrow was displayed. In the RESPOND task participants only responded when they were presented with an up or down arrow by indicating the direction of the previous left or right arrow. The COMPLEX task was identical to the RESPOND task, except that a dual button press was made in response to down arrows. Figure 2: Task design. Frequent left and right arrows were displayed with a variable interstimulus interval (1,600, 1,700, 1,800, 1,900 or 2,000 ms). In 91 trials, an infrequent up or down arrow interrupted the frequent stimuli at an unpredictable offset (mean=323 ms, s.d.=122 ms). Each task consisted of 4 × 3 min blocks interleaved with 5 × 40 s of rest. This mixed block-event-related design allowed sustained task-rest activations and transient activations during infrequent−frequent stimuli to be estimated separately. In the MONITOR task, individuals responded to frequent stimuli with a corresponding left or right button press. Participants were instructed to simply monitor the infrequent stimuli. In the INHIBITION task, participants were instructed to respond as fast as they could to the left and right arrows but to try and cancel their response if an up or down arrow was displayed. In the RESPOND task participants only responded when they were presented with an up or down arrow by indicating the direction of the previous left or right arrow. The COMPLEX task was identical to the RESPOND task, except that a dual button press was made in response to down arrows. Full size image Behavioural results Results from the four SST variants were analysed using response times (RTs) and accuracy measures. In the MONITOR task, participants responded to frequent left and right arrow cues with a corresponding button press. Infrequent up and down arrow cues, which appeared at a brief variable offset after the frequent cues, were monitored but did not trigger any change in motor response. Errors were defined as the total number of incorrect button presses. Participants had a low failure rate (2.4%, s.d.=1.7%) and rapid RT (median=0.43 s, s.d.=0.06). In the INHIBITION task, participants tried to cancel the frequent left or right responses when presented with the infrequent cues [13] , [35] . Errors were defined as the number of instances in which the participant failed to withhold a button press. Participants showed a high failure rate (54%, s.d.=15.8), which accorded closely with the ~\n50% failure target of titrated SST designs [19] . The mean RT on go trials was longer (median=0.69 s, s.d.=0.19). In the RESPOND task, participants only made a button press when an infrequent cue was detected [6] . Errors were defined as the sum of misses and incorrect responses. There was a low failure rate (4.6%, s.d.=10.4) and a fast RT (median=0.45 s, s.d.=0.06). The COMPLEX task was identical to the RESPOND task, except that the down cue triggered an additional concurrent button press [36] . Errors were defined as the sum of responses, indicating the incorrect direction, misses and failure to press the concurrent button. There was a low failure rate (6.1%, s.d.=5.5) and a long RT (median=0.63 s, s.d.=0.07 NB—calculated from the time of the first button press). Pairwise comparisons of median RTs revealed that the MONITOR and RESPOND tasks did not differ significantly, and the INHIBITION and COMPLEX tasks did not differ significantly (both P >0.2). All other comparisons were significant at P <0.001 two tailed ( Fig. 3a ). 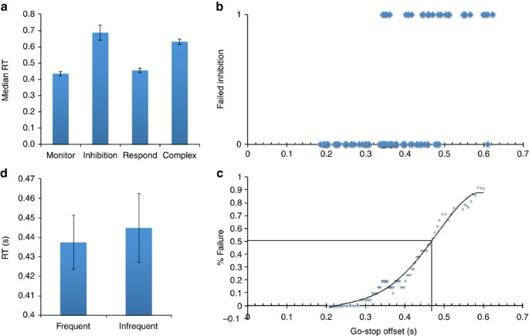Figure 3: Behavioural results. (a) Median RTs were significantly slower for the INHIBITION and the COMPLEX tasks. (b) Representative example of the distribution of successful and failed inhibition trials according to go-stop offset. (c) Calculating the point at which the individual inbfailed 50% of the stop trials. (d) There were no significant RT costs during the MONITOR task when infrequent stimuli were detected despite there being high levels of activation within the right inferior frontal cortex. All error bars report s.e.m.,N=16. Figure 3: Behavioural results. ( a ) Median RTs were significantly slower for the INHIBITION and the COMPLEX tasks. ( b ) Representative example of the distribution of successful and failed inhibition trials according to go-stop offset. ( c ) Calculating the point at which the individual in b failed 50% of the stop trials. ( d ) There were no significant RT costs during the MONITOR task when infrequent stimuli were detected despite there being high levels of activation within the right inferior frontal cortex. All error bars report s.e.m., N =16. Full size image Functional topography of the right lateral frontal cortex We first conducted spatial independent components analysis (ICA) on the activation time courses of voxels within an anatomically defined mask that included the right lateral frontal cortex and insula. Calculation of the Akaike Information Criteria resulted in seven significant spatial components (C1–C7, Fig. 4 and Table 1 ). C2 was centred on the anterior insula/inferior frontal operculum (AIFO), near the expected location of the putative reactive inhibition module. C4 was located within the posterior lateral orbitofrontal cortex (pLOFC), also a probable candidate for a reactive inhibition module. C7 was located within the IFS and was a probable candidate for the proactive inhibitory module [6] , [29] . The other four components were located within the anterior lateral orbitofrontal cortex (C1—aLOFC), the superior frontal sulcus (C3—SFS), the lateral frontal polar cortex (C5—FPC) and the rostrolateral frontal cortex (C6—RLFC). Five-millimetre radius spherical region of interest (ROI) were defined at the peak coordinates of all seven components for further analysis. 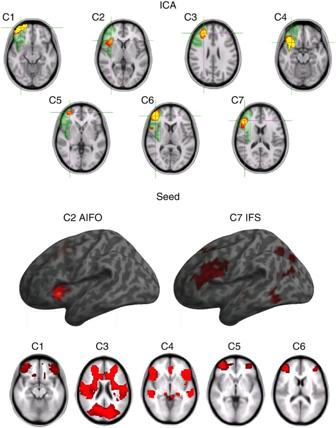Figure 4: ICA and seed analysis. (Upper) Seven components from the ICAs. C2 corresponded closely to the expected coordinates of the right anterior insula/inferior frontal operculum (AIFO). C7 corresponded closely to the expected coordinates of the RIFS. The other five components were within: C1—anterior lateral orbitofrontal cortex (aLOFC). C3—superior frontal sulcus (SFS), C4—posterior lateral orbitofrontal cortex (pLOFC), C5—frontopolar cortex (FPC) and C6—rostrolateral prefrontal cortex (RLFC). (Lower) Each of the regions identified by the ICA of the right frontal cortex was associated with a larger-scale network that included bilaterally distributed cortical regions. Notably, the C2 and C7 networks conformed closely to the ‘working memory’ and ‘reasoning’ networks that were reported in another recent study29. Figure 4: ICA and seed analysis. (Upper) Seven components from the ICAs. C2 corresponded closely to the expected coordinates of the right anterior insula/inferior frontal operculum (AIFO). C7 corresponded closely to the expected coordinates of the RIFS. The other five components were within: C1—anterior lateral orbitofrontal cortex (aLOFC). C3—superior frontal sulcus (SFS), C4—posterior lateral orbitofrontal cortex (pLOFC), C5—frontopolar cortex (FPC) and C6—rostrolateral prefrontal cortex (RLFC). (Lower) Each of the regions identified by the ICA of the right frontal cortex was associated with a larger-scale network that included bilaterally distributed cortical regions. Notably, the C2 and C7 networks conformed closely to the ‘working memory’ and ‘reasoning’ networks that were reported in another recent study [29] . Full size image Table 1 Peak coordinates from the ICA of right frontal cortex. Full size table Unique modules versus distributed networks Activation time courses were extracted from the seven ICA ROIs for each task and each participant. These ‘seed’ time courses were entered into a general linear model (GLM) with voxel time courses as the dependent variables. Contrast images were generated that averaged across the four tasks and the resultant seven whole-brain maps were examined at the group level using repeated measures analysis of variance (ANOVA) in SPM8. Consistent with the ARP model [29] , when the right AIFO seed was contrasted against the other six seeds [37] , significantly greater functional connectivity was evident across a bilateral network, including the left AIFO and the anterior cingulate cortex (ACC)/preSMA ( Fig. 4 and Supplementary Table 1 ). Similarly, when the right IFS seed was contrasted against the other six seeds, significantly greater functional connectivity was evident across a bilateral network, including the left IFS and the inferior parietal cortices. Contrasting the other five seeds in a similar manner generated five more distributed functional networks. Reactive inhibition versus infrequent cue detection To test the hypothesis that an IFG sub-region is specialized to reactive inhibition, transient activations in response to infrequent cues were compared across the four SST variants using ANOVA in SPM8. The positive effect of condition (T-contrast collapsing across all four SST variants) revealed transient increases in activation in response to infrequent cues within all seven ICA ROIs ( Table 2a ). There were no significant main effects of Task. Contrasting the INHIBITION minus the MONITOR task showed no significant effects in any of the ROIs ( Table 2b ). Similarly, contrasting the INHIBITION task minus all other tasks showed no significant effects ( Table 2c ). Contrasting the COMPLEX task minus the MONITOR task also showed no significant effects ( Table 2d ). When whole-brain voxel-wise analyses were conducted, no voxels within the frontal lobes showed a main effect of task (that is, differences between the four variants) even when applying a liberal uncorrected threshold of P <0.01 one tailed. There was a strong positive effect of condition within the RIFC at the whole-brain-corrected threshold ( Fig. 5a ). The RIFC was not unique in its sensitivity to infrequent cues; activation clusters were also evident within other regions of the right lateral frontal cortex, and more broadly within the left lateral frontal cortex, parietal cortices bilaterally, the preSMA and ACC. Thus, IFC regions were sensitive to the presentation of infrequent cues but were insensitive to motor inhibition demands [13] , [17] , [21] . Table 2 ROI analysis of transient activations. 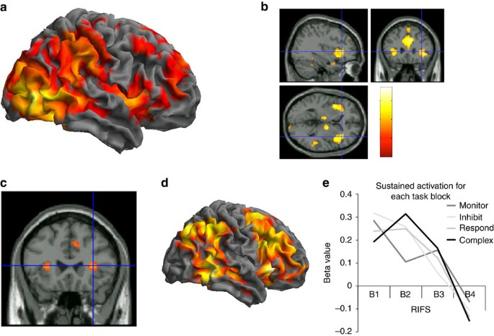Figure 5: Within-subject fMRI results. (a) When examining the response to infrequent stimuli collapsed across the four tasks, robust transient activation was evident within a set of brain regions that included inferior frontal cortex. However, this activation was no greater in the INHIBITION variant of the task (tcontrast whole-brain FDR-corrected atP<0.05). (b) Activation within the AIFO bilaterally, the ACC and preSMA was greater for failed relative to successful inhibition trials (tcontrast rendered atP<0.01 uncorrected for display purposes). (c) The AIFO bilaterally, the ACC and preSMA were the only frontal-lobe regions to show significantly greater sustained activation when contrasting task blocks versus rest blocks (tcontrast whole-brain FDR-corrected atP<0.05). (d,e) A set of brain regions including the right AIFO and the right IFS were strongly activated in the early blocks, when learning was maximal relative to the late blocks, when responses were established (tcontrast whole-brain FDR-corrected atP<0.05). No frontal lobe areas showed heightened activation during late blocks relative to early blocks when applying a liberal uncorrected threshold ofP<0.01. Full size table Figure 5: Within-subject fMRI results. ( a ) When examining the response to infrequent stimuli collapsed across the four tasks, robust transient activation was evident within a set of brain regions that included inferior frontal cortex. However, this activation was no greater in the INHIBITION variant of the task ( t contrast whole-brain FDR-corrected at P <0.05). ( b ) Activation within the AIFO bilaterally, the ACC and preSMA was greater for failed relative to successful inhibition trials ( t contrast rendered at P <0.01 uncorrected for display purposes). ( c ) The AIFO bilaterally, the ACC and preSMA were the only frontal-lobe regions to show significantly greater sustained activation when contrasting task blocks versus rest blocks ( t contrast whole-brain FDR-corrected at P <0.05). ( d , e ) A set of brain regions including the right AIFO and the right IFS were strongly activated in the early blocks, when learning was maximal relative to the late blocks, when responses were established ( t contrast whole-brain FDR-corrected at P <0.05). No frontal lobe areas showed heightened activation during late blocks relative to early blocks when applying a liberal uncorrected threshold of P <0.01. Full size image Successful inhibition versus error detection To test the hypothesis that successful inhibition results from a stronger inhibitory signal [19] , infrequent trials from the INHIBITION task were subdivided into those in which the participant successfully cancelled their response (SUCCESSFUL) and those in which the motor response was completed (FAILED). Contrasting activations related to SUCCESSFUL and FAILED inhibition trials showed the opposite effect from that predicted by the RIPI model, with greater activation for unsuccessful trials in the pLOFC and the AIFO ROIs ( Table 2e ). Unconstrained voxel-wise whole-brain analyses also showed no significant voxels within the IFC when contrasting SUCCESSFUL minus FAILED inhibition trials with a liberal uncorrected threshold of P <0.01 one tailed; however, the reverse contrast revealed bilateral activations centred around the AIFO, ACC and preSMA ( Fig. 5b ). These results accord with a more general role for IFC in attention, the focus of which is likely to be captured when erroneous responses are detected [6] , [8] , [38] , [39] . Proactive inhibition versus rule processing Sustained task versus rest activations were examined using ANOVA with the factor Task to determine whether the IFS was sensitive to proactive inhibition demands. The positive effect of condition showed significant sustained activation in the right AIFO ROI but not within the IFS or any other ROIs ( Table 3a ). Contrasting sustained activation during the INHIBITION task relative to the MONITOR task did not show significantly greater activation in any of the ROIs ( Table 3b ). Similarly, contrasting the INHIBITION task relative to the mean of the other three tasks did not show increased activation ( Table 3c ). Contrasting sustained activation during the COMPLEX minus the MONITOR task showed significantly greater activation in the RIFS ( Table 3d ). Similarly, contrasting the COMPLEX minus the INHIBITION task showed significant effects within the RIFS, the FPC and the aLOFC ROIs ( Table 3e ). However, contrasting the COMPLEX minus RESPOND task did not generate a significant result. Unconstrained voxel-wise analyses produced a similar pattern of results. The positive effect of condition rendered significant activation across a bilateral set of brain regions, including AIFO and the ACC, and supplementary motor area ( Fig. 5c ). There were no significant areas of activation within the IFS or within more anterior frontal lobe regions at the liberal uncorrected threshold of P <0.01 one tailed. Nor were there any significant voxels within the frontal lobes when contrasting the INHIBITION task minus the MONITOR task or when contrasting the INHIBITION task minus the other three SST variants. Contrasting the COMPLEX minus the MONITOR or INHIBITION tasks also showed no significant effects within the frontal lobes at the uncorrected threshold. These results provide modest evidence in support of a role for the IFS in processing more complex sets of stimulus–response rules and suggest that general preparatory processes engage the AIFO network. Table 3 Regions of interest analysis of sustained activations. Full size table Response inhibition versus the learning of novel tasks According to the RIPI hypothesis, inhibitory modules within the IFC work to downregulate routine behaviours [17] , [21] . Consequently, inhibitory neural modules should be less active at the beginning of the SST, when frequent responses are yet to become routine. Conversely, the ARP model proposes that the AIFO and IFS are involved during tasks that tax attention and that involve processing novel or complex rules, respectively. These latter classes of processes should be greatest towards the beginning of a task, when new behaviours are being established [38] , [40] . To test between these predictions, the fMRI data were remodelled with four sustained predictor functions per task, one for each block of task acquisition. When activations were examined using 4 × 4 full factorial models with the factors Task and Block, the results supported the ARP as opposed to the RIPI hypothesis. Specifically, contrasting early versus late blocks (B1=2, B2=1, B3=−1, B4=−2) showed stronger activation within all seven ICA ROIs ( Table 4a ) with no significant Task × Block interactions. Similarly, all seven ROIs were more active in early relative to late blocks when analysing the INHIBITION task alone ( Table 4b,c ). Unconstrained voxel-wise analyses produced a similar result. When early (less familiar) blocks were subtracted from late (more familiar) blocks (B1=−2 B2=−1 B3=1 B4=2), no significant voxels were rendered within the frontal lobes ( P <0.01 uncorrected and one tailed) nor were regions evident when the contrast was repeated for the INHIBITION task alone. Contrasting early minus later blocks (B1=2 B2=1 B3=−1 B4=−2) rendered extensive clusters across the frontal and parietal cortices ( Fig. 5d,e ) at the whole-brain-corrected threshold. There was no significant interaction between Task and Block, and no main effect of Task. Table 4 Regions of interest analysis of task familiarity effects. Full size table Psychophysiological interactions According to the RIPI model, a ‘hyperdirect pathway’ between the right IFC and the sub-thalamic nucleus (STN) works as a brake on the motor system during reactive inhibition [12] . To test this hypothesis, the AIFO was used as a seed region in PPI analyses, which identified brain areas where the activation time course was more correlated with the seed region during infrequent relative to frequent cues [41] . Whole-brain maps depicting β-weights for the PPIs were examined using ANOVA with Task as the factor. The positive effect of condition showed a strong PPI within predefined STN ROIs bilaterally and within the three sensorimotor cortex ROIs ( Supplementary Table 2a ); however, there was no significant main effect of task ( Supplementary Table 2b ). Numerically, the greatest STN PPI was for the RESPOND task not the INHBITION task. A second analysis examined the PPI within the other six ICA ROIs. The superior frontal sulcus, pLOFC and rIFS all showed significantly greater correlations with the AIFO time course during infrequent relative to frequent cues and no significant main effects of task. Contrasting the PPI for the INHIBITION task minus the MONITOR task did not generate any significant differences. Similarly, the voxel-wise whole-brain analysis showed no significant main effect of task at the corrected (false discovery rate (FDR), P <0.05) threshold. Analysis at the liberal uncorrected threshold of P <0.01 rendered several clusters within the frontal and parietal cortices; however, although many of these regions did show heightened PPI for the INHIBTION task, they also showed heighted PPI for the COMPLEX task, in which the routine response was not cancelled ( Supplementary Fig. 1 ). Repeating the PPI analysis with the pLOFC as the seed region also generated no significant main effects of Task on the PPI for STN and motor ROIs (all P >0.3). Similarly, when the magnitudes of activation within the STN ROIs were examined for the transient ANOVA reported above, there was a significant positive effect of condition (left t =3.44, P <0.001; right t =2.51, P <0.01) but no significant main effect of task (left F=2.21, P =0.096; right F=0.85, P =0.470). Because of the small size of the STN and its variable anatomical location, we repeated our analyses using individually defined ROIs drawn on high-resolution structural scans (see Methods); the same result was evident when using this approach (positive effect of condition t =1.95, P =0.035 main effect of task, P >0.3). Individual differences analyses The RIPI model predicts that individual differences in the functioning of a RIFG module uniquely contribute to between-subject variability in reactive inhibition performance. To test this hypothesis, we calculated each individual’s stop signal reaction time (SSRT): this being the time required to cancel a routine response (mean SSRT=181 ms, s.d.=106 see Methods and Fig. 3b ). We first tested the prediction that the magnitude of activation within the IFC ROIs would correlate negatively with SSRT. Contrary to some prior studies [42] , we observed no significant negative correlations ( Supplementary Table 3a ); unexpectedly, there was a significant positive correlation with transient activation on reception of infrequent cues within the right pLOFC. We then tested whether individual differences in SSRT relate to the functional connectivity between the RIFC and motor processing areas. Individual variability of PPIs seeded with right AIFO were examined for the INHIBITION task using a repeated measures ANOVA with the within-subject factor target ROI (3 × motor ROIs and 6 × RIFC ICA ROIs) and SSRT as a covariate. There was a significant effect of SSRT (F(1,14)=10.894, P <0.005) with no main effect of ROI and no interaction (both P >0.1). Bivariate correlations demonstrated significant negative correlations with SSRT not only in the motor ROIs but also in RIFC ROIs ( Fig. 6 and Supplementary Table 3b ). This effect was not specific to the right AIFO because when the analysis was repeated seeding by the left AIFO, ANOVA again revealed a significant effect of SSRT (F(1,14)=4.94, P =0.043). There was also a main effect of ROI (F(8,112)=2.45, P =0.017) and an interaction between SSRT and ROI (F(8,112)=2.54, P =0.014. These effects were driven by significant negative correlations with SSRT in the aLOFC, pLOFC and one motor cortex ROI, and sub-threshold trends in the FPC, pre Motor Cortex (PMC) and the other two motor cortex ROIs. Similarly, when the ACC/preSMA was used as a seed region, there was a significant effect of SSRT (F(1,4)=4.92, P =0.043) with no significant main effect of ROI or ROI × SSRT interaction (both P >0.3). Thus, reactive inhibition performance related to the interactions of multiple distributed functional networks as opposed to a specific frontal–posterior functional connection. 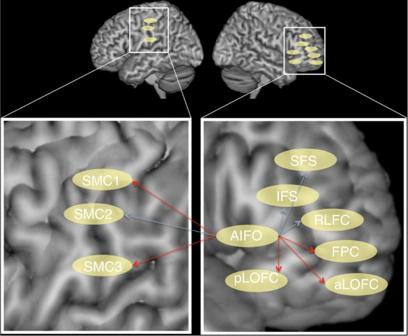Figure 6: Individual differences analysis. The INHIBTION task showed significant correlations (N=16) between SSRT and the infrequent–frequent PPIs across many of the ICA and SMC ROIs when seeded with the right AIFO ROI time course. Similar results were evident when seeded with the right pLOFC, the ACC/preSMA and the left AIFO demonstrating that behavioural inhibition is related to a broad graph of inferior frontal cortex connections. Significant PPIs are indicated by red arrows. Figure 6: Individual differences analysis. The INHIBTION task showed significant correlations ( N =16) between SSRT and the infrequent–frequent PPIs across many of the ICA and SMC ROIs when seeded with the right AIFO ROI time course. Similar results were evident when seeded with the right pLOFC, the ACC/preSMA and the left AIFO demonstrating that behavioural inhibition is related to a broad graph of inferior frontal cortex connections. Significant PPIs are indicated by red arrows. Full size image The results presented here are consistent with those of previous studies insofar as they demonstrate that right IFC sub-regions are strongly activated during performance of a classic inhibitory control paradigm. Furthermore, they confirm the significant relationship between IFC functional activation and inhibitory task performance. However, they also highlight how the hypothesis of unique inhibitory modules within the frontal lobes is inaccurate in at least seven important respects. First, although several IFC regions showed transient activations during motor inhibition, equivalent effects were observed during the three control tasks, all of which had minimal inhibition demands. Second, there was no evidence of greater activation within the right IFC during successful minus unsuccessful inhibition. Instead, the opposite effect was evident in the AIFO and the pLOFC. Third, counter to the notion of a module for proactive inhibition [17] , there was no evidence of sustained proactive activation in the right IFS during the INHIBITION task. Indeed, on average, there was no sustained IFS activation relative to rest. Instead, the AIFO–ACC network showed significant sustained task-related activation and this activation was not disproportionately strong during the INHIBITION task. Fourth, IFC sub-regions were particularly active in the initial blocks of the INHIBITION and the control tasks as opposed to in the final block of the INHIBITION task when established responses had to be overridden; a result that accords closely with other recent findings [30] , [43] of a general attentional role for the AIFO–ACC network, and that supports the view that frontoparietal regions in general are strongly recruited during the learning of novel tasks as opposed to when inhibiting dominant behaviours. Fifth, the results of the data-driven ICA analyses accorded poorly with the hypothesis of functionally unique modules within the IFC [1] , [17] . More specifically, each activation time course from the sub-regions identified in the ICA of right IFC correlated with a distributed cortical network [33] and none of the right IFC sub-regions were unique in their sensitivities to task manipulations. Sixth, although functional connectivity from right IFC to STN was greater during inhibition than go trials, similar effects were observed for the non-inhibitory task contexts and for functional connectivity between other frontal lobe regions. Finally, the individual differences analyses of functional connectivity strengths demonstrated that individual motor inhibition performance relates to a family of within- and between-network interactions as opposed to any single frontal–posterior connection [12] , [34] . Based on these results, it is reasonable to conclude that reactive inhibition and proactive inhibition are two specific examples of the wide range of cognitive demands that are supported by domain general frontal–parietal networks [6] , [7] , [24] , [25] , [29] . One objection could be that the IFC is an extensive anatomical structure that houses multiple functionally distinct sub-regions. Perhaps the current study focused on the wrong set of IFC sub-regions and, consequently, inhibitory modules may yet exist in other areas that were not analysed? In fact, several authors have suggested that a better functional subdivision of IFC should be established [33] , [44] , [45] , [46] . Moreover, it has been proposed that the reactive inhibition module is located at the most posterior and lateral extent of the inferior frontal gyrus as opposed to within the AIFO [17] , [36] , [47] . However, although the ICA identified multiple components within the IFC, none of them responded significantly more to infrequent cues in the INHIBITION relative to the control tasks; yet, several of these ROIs were related to inhibitory task performance as gauged by correlations between SSRT and functional connectivity measures. Furthermore, when supplementary voxel-wise analyses were run with a liberal uncorrected threshold, no voxels within the right IFC showed a disproportionately strong response in the INHIBITION task. Indeed, we could find no evidence of an inhibitory module anywhere within the frontal lobes. Thus, the likelihood of a reactive inhibition module being overlooked is vanishingly small. Another potential objection could be that the infrequent cue conditions from the control tasks might have tapped ‘hidden’ inhibitory demands. Perhaps, simply engaging in a task or processing an infrequent stimulus engages the top-down inhibition of other distracting information. From this perspective, one would expect to see transient IFC activation to stimuli in all four SST variants [48] . This objection provides a poor account of the results observed here for several reasons. Monitoring for infrequent cues was the central aim for participants in all four SST variants and, consequently, their presentation once in every four trials was anticipated as opposed to surprising. Indeed, we have previously reported that target stimuli elicit significantly greater right IFC activation than distractors even when they are presented at the same frequency [28] . Furthermore, it has been stated that the inhibitory role of the RIFG is evidenced by the reflexive slowing of all motor processes on reception of infrequent events [48] ; however, in the MONITOR task, there was no significant increase in RT during trials that were interrupted by the presentation of infrequent cues ( t =1.035, P =0.16 one tailed Fig. 3d ) despite the fact that the AIFO and pLOFC ROIs were activated to the same level as during the INHIBITION task. More importantly, even if attention to task did involve some level of top-down inhibition, from the RIPI perspective a task that has the same stimulus presentation parameters but which also involves overriding a dominant motor response should require significantly more top-down inhibition. Yet, we observed no greater activation or functional connectivity for RIFC sub-regions during the INIHBITION task. This latter point highlights a salient theoretical issue regarding the literature on inhibition, which is that behavioural inhibition and neural inhibition are often conflated. The former refers to the effortful cancellation of a dominant behaviour, whereas the latter refers to the suppression of neural firing. We would argue that although this conflation is intuitively attractive it is also over-simplistic and computationally unrealistic. Neural inhibition is a pervasive property of systems throughout the brain and is critical for a raft of processes that are not considered part of a behavioural inhibition construct. Moreover, neural inhibition can work at multiple scales, including large-scale systems and local lateral connections [7] . At the large scale, one neural system, for example, a network or a module, may be negatively coupled with another. A prominent example is the robust negative correlation that is observed between the Default Mode Network and active state networks [49] . The popular systems level account of behavioural inhibition states that there is a ‘hyperdirect pathway’ [12] , [50] , [51] between the IFC and the STN. Specifically, the reactive inhibition module is posited to upregulate activity within the STN via a fast hyperdirect connection. In response, the STN works as a brake by exercising neural inhibition over motor systems. Models such as the hyperdirect pathway are attractive in their simplicity and seem plausible when one considers the well-established role of the STN in motor dysfunction [52] . However, the results of the current study fit poorly with the idea that a hyperdirect pathway is specifically or even particularly involved in systems level inhibition. For example, although the PPI analyses showed an increase in connectivity from the AIFO to the STN and SMC ROIs during motor inhibition, this heightened connectivity was largest in the RESPOND task. Therefore, if there is a hyperdirect pathway, it is also involved in more general motor control. It should be noted that fine-grained control also does not require top-down inhibitory signals. This is because lateral inhibition is a common property of neural systems on the local level. Lateral inhibition allows alternative representations within the same neuronal population to compete for limited processing resources while helping to maintain computationally important properties of neural networks such as pattern separation and representation stability. A consequence of lateral inhibition is that if top-down potentiation specifically targets one representation, it will lead to the lateral suppression of other competing representations [53] and the slowing of concurrent processes. Herein lies a problem for the hypothesis of unique inhibitory modules within the brain; the prevalence of lateral inhibition in the context of top-down potentiation renders specialized modules that output inhibitory signals redundant. Indeed, from a computational perspective, top-down potentiation mechanisms are more efficient than top-down inhibitory mechanisms. Consider the processing of a sequence of task relevant stimuli against a background of noise in the form of changing distractors. To prevent task processes from being disrupted, the source of a top-down inhibition signal would be required to represent and downregulate each distracting item individually. This representation of distractor items would be prone to error because it would have to be continually maintained, monitored, updated and extended. By contrast, the source of a top-down potentiating signal could maintain and upregulate just those items that were relevant to the task at hand. Lateral inhibition would inhibit other competing processes regardless of their exact pattern of representation. Given the computational advantages of top-down potentiation, it is unsurprising that electrophysiology research has provided a wealth of evidence, demonstrating that lateral frontal cortical neurons represent task-relevant inputs, rules and responses [54] , [55] , [56] . This same basic top-down potentiation mechanism is theoretically able to support a range of general cognitive phenomena, including inhibition, attention and working-memory maintenance. These phenomena fit closely with the broad set of conditions that recruit the AIFO–ACC network. For example, in a recent study, lateral frontal and inferior parietal brain regions were analysed using an ICA of task versus rest activation patterns from 12 different cognitive paradigms. In that study, highly similar AIFO and IFS networks were observed to those reported here [29] . The AIFO–ACC network was recruited across almost all task contexts; however, activation was greatest during the working memory tasks, which required information to be maintained in mind over a delay. This network was statistically similar to that which is observed during target detection. Consequently, the AIFO–ACC network’s activation profile makes it a strong candidate for a top-down potentiation source. In the same study [29] , the IFS network was particularly active during tasks that required more complex cognitive processes, for example, reasoning, planning and mental rotation. More broadly, the IFS is particularly closely associated with tasks in which information has to be transformed as opposed to simply maintained in mind. For example, when processing verbal [30] and non-verbal reasoning problems [31] , and when the contents of working memory are reorganized [57] . Consistent with these observations, the IFS was the only ROI to show heightened activation during the COMPLEX task. The fact that this effect was small is likely to be a consequence of the rule-processing demands in the current study being modest relative to a challenging reasoning or planning task. This study has a number of limitations and raises several important questions for future investigation. One of the reviewers commented that the STN is small and anatomically variable, making localization difficult. It should be noted, however, that our spatial smoothing and voxel sizes were matched to those reported in the original article that proposed the hyperdirect pathway between the RIFG and the STN [12] , and we are confident, therefore, that we examined the same functional connection. Nonetheless, a sensible future study would investigate the role of the STN with a similar set of tasks and imaging sequences optimized for the STN, with finer resolution and using physiological monitoring to control for artefacts frequently found in the midbrain. Higher-resolution scanning would allow activation originating from the STN to be more precisely differentiated from other proximal sub-thalamic structures. Another reviewer noted that there were more females than males in the current study. However, we observed no significant male–female difference in RIFG activation in this study, nor did we observe male–female differences in RIFG activation when examining 60 previously collected SST data sets. Consequently, the results are likely to be representative of both males and females. It is also notable that the within-subject and individual differences analyses both point towards an important role for functional connections both within and between networks that come into close proximity in the inferior frontal cortices. We propose that as opposed to arbitrarily focusing on any one task, connection or module [37] a sensible future direction would be to examine the entire graph of local and distal connections that constitute frontal lobe functional architecture in a large-scale cohort and to relate those measures to individual differences in motor inhibition and to cognition more generally. Thus, the question arises of whether impulsivity disorders may be further classified according to the exact functional network or set of functional connections that are affected within this architecture. Such sub-classification of patient populations has the potential to improve clinical outcomes by more accurately guiding the selection of interventions [58] , [59] . Experimental design The four tasks were based on the design reported by Rubia et al. [19] , which in turn is a variant on the paradigm reported by Logan and Cowan [35] . Participants were presented with 342 frequent left and right arrows with an unpredictable interstimulus interval of 1,600, 1,700, 1,800, 1,900 or 2,000 ms ( Fig. 2 ). Infrequent up or down arrow interrupted the presentation of the frequent stimuli in 91 of the trials. Stop signal were presented on average at 323 ms after the frequent signal with an s.d. of 122 ms. These values were selected based on prior data from young controls, indicating that an ~\n50% failure rate should be expected for stop-signal trials with this offset. In the classic SST, participants indicate left or right with a button press when left and right arrows are presented. They are instructed to press the button as quickly as they can but to try to cancel that response if a stop signal is presented. Here, participants undertook four novel variants of the classic SST. The variants were precisely matched with each other in terms of the rate and frequency of stimulus presentation. However, stimulus delivery differed from the classical task in three key respects. First, the classical SST does not allow sustained activation during routine responding to be estimated using fMRI, because these responses are too frequent to reliably estimate relative to the constant term of the GLM. To measure activation related to proactive inhibition, it was necessary to compare variations in sustained activation across task contexts. Consequently, each SST variant was broken down into 4 × 3-min blocks of continuous task performance interleaved with 5 × 40 s of rest. This design enabled the reliable estimation of sustained activity in response to frequent stimuli and transient activation due to infrequent stimuli. Thus, the tasks were undertaken in separate scanning acquisitions with four blocks of task interspersed with rest periods. The order in which the tasks were undertaken was inverted in half of the participants to average out differences in stimulus familiarity across tasks. Second, to allow the complexity of the possible responses to frequent cues to be varied across the four tasks, two alternative stimuli were used, these being an up arrow and a down arrow. These cues were presented pseudo randomly and at approximately equal frequency to each other with the sum of the two frequencies matched to that of stop signals in the classic SST paradigm. Finally, the classic SST and the go-stop inter-stimulus interval is varied dynamically to force participants to a 50% failure rate. This design is intended to keep the task challenging while allowing an estimation of the mean SSRT, this being the amount of time taken for inhibitory processes to override the initiated motor response. Several of the variants applied here did not have an inhibitory requirement. Consequently, the mean go-stop inter-stimulus interval was matched to that from a previous study with controls of similar age distribution [15] and with a variable jitter to make it impossible to predict the exact time of the stop signal on any given trial. It was predicted that failure rates for the stop-signal trials would be ~\n50%. The four tasks were designed to match each other in terms of the visual properties and the structure of the GLM that was used to fit psychological predictor functions to brain activation time courses. The tasks varied with respect to reactive inhibition, proactive inhibition and rule-processing demands. Response requirements for the four tasks varied as follows. 1 MONITOR. Participants made immediate left or right button presses in response to the left and right arrows. They were instructed to monitor the infrequent up ad down arrow cues but to continue responding as per normal with the left and right button press. 2 INHIBITION. Participants made immediate left or right button presses in response to left and right arrows. They tried to cancel those responses on trials that were interrupted by the infrequent up and down arrows but not to slow the initiation of the response (equivalent to classic SST). 3 RESPOND. Participants responded with the left or right button press when the trials were interrupted by up and down arrows. On all other trials, no response was made (equivalent to target detection [26] ). 4 COMPLEX. The same as the RESPOND task, except that when trials were interrupted by a down arrow participants made a dual button press. Thus, a more complex set of stimulus–response rules were to be acquired and processed. Notably, this manipulation involves initiation of an extra response, but does not require the inhibition of a planned response [36] . Participants Sixteen right-handed individuals (5 male, 11 female) between 18 and 25 years of age participated in the study. All participants had normal hearing and corrected to normal vision. Exclusion criteria included a history of neurological or psychiatric illness and individuals taking psychoactive medications. Before commencing the study, participants gave informed consent. The University of Western Ontario Research Ethics Board approved this study 17886E. Data collection Before being scanned, participants read an information sheet detailing the task requirements. Once in the scanner, participants were reminded of the current instructions verbally before each block began. Responses were made using an MRI-compatible button box. The task was displayed on a projector screen at the end of the scanner bore, visible via a mirror placed just in front of the eyes. Brain images were collected using a 3-Tesla Siemens Scanner. 310 T2-weighted echo-planar images depicting BOLD contrast were acquired per block of scanning acquisition. The first ten images were discarded to account for equilibrium effects. Each image consisted of 32 × 3 mm slices, each with a 64 × 64 matrix and a 192 × 192 mm field of view. Images of each participants brain were collected with a 2-s repetition time, a Echo Time of 30 ms, a flip angle of 78°, echo spacing of.51 ms and a bandwidth of 2,232 Hz/Px. Before analysis, the data were pre-processed in SPM8 (Statistical Parametric Mapping, Welcome Department of Imaging Neuroscience, London, UK). Data were slice-timing and motion corrected, spatially normalized to the standard Montreal Neurological Institute template and spatially smoothed with an 8-mm full width at half maximum Gaussian kernel. The data were high-passed filtered (cutoff period=180 s) to remove low-frequency drifts in the MRI signal. First-level fMRI model The fMRI data were modelled at the individual participant level in SPM8. Two predictor functions were generated for each task. The first predictor function was designed to capture sustained activations during routine responding and consisted of the onset and duration times for all frequent and infrequent trials convolved with the canonical haemodynamic response function (HRF). (A frequent trial was defined as the presentation of a left or a right arrow alone and an infrequent trial was defined as the presentation of a left or a right arrow with interruption by an up or a down arrow). The second predictor function was designed to capture transient increases in activation in response to infrequent trials. This latter predictor function consisted of the onsets and durations for all infrequent trials convolved with the HRF, minus the onsets and durations for all frequent trials convolved with the HRF. Noise due to movement was accounted for by inclusion of six nuisance variables for each task acquisition, corresponding to translations and rotations in the x , y and z planes. An additional model was run at the individual participant level, in which the sustained predictor functions were broken down into four task blocks without inclusion of the transient predictor function. In this manner, effects of familiarity and novelty on activation could be examined within and across task. Group-level fMRI analyses Spatiotemporal ICA was carried out using the MELODIC command line function from the FSL toolbox [60] with the concatenate option. The ICA was restricted to an anatomical mask, including the right lateral frontal cortex and insula. The mask was defined by combining regions from the automatic anatomical labelling templates [61] . Whole-brain maps, depicting β-weights for the experimental predictor functions from the first-level models were collated for group-level random effects analyses. Focused ROIs analyses were carried out with the MarsBaR toolbox [62] , which calculates the average value from all voxels within the ROI. Voxel-wise group-level analyses were carried out in SPM8 and, unless reported otherwise, used a FDR correction of P <0.05 for multiple comparisons across the whole-brain volume. Psychophysiological interaction (PPI) analyses were carried out in SPM8 with physiological time courses extracted using the volume of interest function, which extracts the first eigenvector from voxels within the ROI. Motor cortex regions were examined using ROIs from a previous publication that examined SST activation [6] . STN ROIs for the main analyses were based on the activation coordinates reported in the study that proposed the hyperdirect pathway [12] (Montreal Neurological Institute (MNI) space, x =±10, y =−15, z =−5). In the secondary analysis, central STN voxels were defined individually in native space using the higher resolution (1-mm voxel size) structural scans. More specifically, the image was drawn on an axial slice of T1-weighted 1-mm isotropic image. These images are not specifically optimized for visualization of the STN; however, we could identify a hypointense region (on both the axial and coronal slices) bounded by white matter that we identified using the following landmarks based on Lambert et al. [63] . The region was approximately in line with the optic tract in the sagittal plane, it was superior to the substantia nigra in both axial and coronal planes. It was posterior to the grey matter between the mamillothalamic tract and fornix. It was medial to the internal capsule and inferior to the anterior commissure. These native-space ROIs were mapped into MNI space using the same transform from the spatial normalizations stage of pre-processing (mean MNI space, left x =8.1, y =−15.6, z =−6.6; right, x =−6.9, y =−15.6, z =−6.8) ( Supplementary Table 4 reports individual STN coordinates). PPI time courses were generated for each individual and for all four tasks in the following manner. The time courses (first eigenvector) within a 10-mm sphere based at the peak right AIFO activation locus from the ICA was extracted for each task and the neural signal underlying the BOLD response was estimated using deconvolution in SPM8. The estimated neural time course was multiplied with a time course in which trials with infrequent up and down arrows were set to 1 and trials with frequent left and right arrows were set to −1. All other time points (that is, rest) were set to 0. The resultant time course was convolved with the HRF to generate a PPI time course. The physiological, convolved psychological and convolved PPis were fitted to the time courses for each voxel within the brain using a GLM in SPM8. Further PPI analyses repeated this procedure, but using time courses from the left AIFO, the preSMA and the right pLOFC ROI coordinates as seeds. Individual differences analyses examined correlation of activation and functional connectivity measures with the SSRT. The SSRT provides an estimate of the amount of time taken for an individual to cancel an initiated response and is defined as the difference between the average RT on go trials and the go-stop offset at which there is 50% failure to cancel a response. The go-stop offset was calculated as follows: (1) all 91 infrequent cues from the INHIBITION task were ordered according to go-stop offset. (2) The percentage failure rate was calculated using a sliding window consisting of 21 trials centred from position 11 to 81. (3) A curve was fitted to the data and the go-stop offset calculated as the point at which the curve crossed the 50% line. Figure 3b,c provides a representative. ANOVAs and non-parametric correlations were carried out in SPSS and used the data extracted via MarsBaR, from the within-subject analyses that were reported in previous sections of this paper. How to cite this article: Erika-Florence, M. et al. A functional network perspective on response inhibition and attentional control. Nat. Commun. 5:4073 doi: 10.1038/ncomms5073 (2014).